Biting disrupts integration to spur skull evolution in eels The demand that anatomical structures work together to perform biological functions is thought to impose strong limits on morphological evolution. Breakthroughs in diversification can occur, however, when functional integration among structures is relaxed. Although such transitions are expected to generate variation in morphological diversification across the tree of life, empirical tests of this hypothesis are rare. Here we show that transitions between suction-based and biting modes of prey capture, which require different degrees of coordination among skull components, are associated with shifts in the pattern of skull diversification in eels (Anguilliformes). Biting eels have experienced greater independence of the jaws, hyoid and operculum during evolution and exhibit more varied morphologies than closely related suction feeders, and this pattern reflects the weakened functional integration among skull components required for biting. Our results suggest that behavioural transitions can change the evolutionary potential of the vertebrate skeleton by altering functional relationships among structures. The functional relationships among morphological structures are central to understanding the astonishing variety of forms across the tree of life. Complex organisms are made up of suites of structures that interact dynamically during execution of functions essential to meeting life’s demands [1] , [2] , [3] , [4] , [5] . 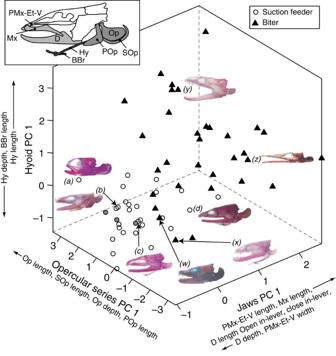Figure 1: Mechanical unit morphological space for 59 anguilliform and 3 other elopomorph species. Axes are the first PCs of phylogenetically controlled interspecific correlation matrices within mechanical units. Axis labels describe the direction of loadings for the morphological variables. Biting species are black triangles and suction feeders are circles; white circles are eels and grey circles are non-anguilliform elopomorphs. Skull images, which have been scaled to the same geometric mean skull size, display a sample of diversity of suction feeding (a–d) and biting species (w–z) across this morphospace. Skulls have been cleared and stained for bone (red) and cartilage (blue). Species identities are as follows: (a) Heteroconger hassi, (b)Conger myriaster, (c)Anguilla japonica, (d)Ophichthus zophochir, (w)Bathyuroconger vicinus, (x)Morigua javanica, (y)Gymnothorax kidako, (z)Oxyconger leptognathus. Inset shows bones of the jaws (light grey shading), hyoid (dark grey) and opercular series (intermediate grey) on a line drawing of anAnguilla rostrataskull. Abbreviations of bone names are as follows: D, dentary; Mx, maxilla; PMx-Et-V ,premaxillo-ethmo-vomer; BBr, basibranchial; Hy, hyoid; Op, opercle; POp, preopercle; SOp, subopercle. For example, the bones of the skull (structures) of teleost fish move in a rapid and highly coordinated manner to expand the mouth cavity and generate suction (function), which they use to capture prey (biological demand; see Table 1 for definitions of key terms). Overlap among structures in function creates dependence, known as functional integration, which can shape the potential for morphological differences to evolve [6] , [7] . Shared genes and developmental pathways can bias the kinds of new phenotypic variants that arise by mutation [8] , [9] , [10] , [11] , [12] , but the resulting combinations of structures must be able to execute their shared function [1] , [2] , [3] , [4] , [6] , [7] (for example, a change in the shape of the hyoid must allow for proper orientation with the jaws and operculum to maintain effective oral expansion). Therefore, functional integration imposes internal selection on morphological variety, culling forms that impair function [7] , [8] , [13] and leading to selective covariance among traits [14] . As this internal selection acts within the organism itself, it can be independent of environmentally imposed selection and is thought to be an important force in the maintenance of morphological similarity among species despite ecological divergence [2] , [3] , [4] . Table 1 Definitions of key terms with examples from this study. Full size table How does diversity arise then, if shared function constrains morphological evolution even in the face of divergent environmental selection? One hypothesis is that the strength of functional integration is not static and can itself evolve [3] , [4] . A number of evolutionary innovations are thought to weaken functional integration among structures. These include the emergence of redundant function in non-overlapping sets of structures [15] , [16] , structural duplication [17] , [18] , [19] , [20] , mechanical decoupling [18] , [19] , [21] and, similar to what we describe here, behavioural transition (also referred to as functional transition), which is a shift in one or more of the functions executed to meet a biological demand. Each of these innovations can break up ancestral functional relationships among structures and permit new trait combinations to arise without disrupting the ability to meet a biological demand. The origin of one of these integration-disrupting innovations may therefore act as a catalyst of morphological diversification, allowing structures to evolve independently of one another, to accumulate differences among species at a faster rate and to reach more extreme forms [1] , [3] , [4] , [15] , [17] . Few empirical studies, however, have connected such innovations—and their associated changes in the strength of functional integration—with shifts in evolutionary integration (that is, correlations between evolutionary change in structures or suites of structures [9] , [11] ), rates of evolution and morphospace occupation (but see related studies by Monteiro et al . [22] and Claverie and Patek [23] ). One of the most prominent and intriguing behavioural transitions in vertebrates is the shift from using suction to directly apprehending prey in the jaws (that is, biting) during aquatic feeding. Delivering a forceful bite is a widespread prey-capture strategy in terrestrial vertebrates, but in aquatic environments biting is relatively rare. Instead, most aquatic feeding vertebrates, including the vast majority of bony fishes, capture prey by suction feeding, which requires tightly coordinated movements of cranial skeletal elements to rapidly increase the volume of the mouth cavity and generate a flow of water strong enough to carry prey into the mouth [24] , [25] , [26] , [27] , [28] , [29] . Aquatic prey capture by biting, on the other hand, entails variable jaw movements that require little to no coordination with other parts of the skull [30] , [31] , [32] , [33] , [34] . Transition from suction feeding to biting is known to involve relaxation of functional integration; however, the evolutionary consequences of shifts in feeding behaviour have never been explored. Here we ask whether the emergence of biting prey-capture behaviour in fishes alters the potential for biting species to diversify in skull morphology compared with closely related species that suction feed. Eels (Anguilliformes) provide an ideal system to investigate this question. With more than 800 species, they make up the vast majority of species diversity of Elopomorpha, a major clade of teleost fishes. Non-anguilliform species of elopomorphs (bonefish, ladyfish and tarpon), similar to most other teleosts, expand their oral cavities to suction feed [24] , [25] , [26] . However, Anguilliformes includes both suction feeders and species that apprehend prey in their jaws by biting [34] , [35] . We hypothesized that the origin of biting released constraints on morphological diversification imposed by the functional integration required to suction feed. We tested three predictions: (1) biting lineages experience weaker evolutionary integration of the skull than suction feeders, (2) weaker evolutionary integration in biters permits accelerated rates of diversification of skull components and (3) biting species exhibit greater morphological disparity (a measure of morphospace occupation) than suction feeders. We collected morphological data for cranial skeletal elements and information on feeding mode, and combined these data with reconstructions of species’ phylogenetic relationships. To test our predictions, we fit evolutionary models that allow biting and suction feeding lineages to differ in the correlations between and rates of diversification within different aspects of the cranial skeleton [36] . We find that components of the feeding mechanism evolve with greater independence in biting eels and this weakened evolutionary integration allows biters to take on a greater variety of morphological combinations compared with suction feeders. These results support our hypothesis that functional integration required for suction feeding constrains skull evolution but transition to biting relieves these constraints. Moreover, our study provides empirical support for the long-standing hypothesis that the strength of functional integration can shape evolutionary integration and the potential to diversify. Evolutionary history of prey-capture behaviour Biting arose within the Anguilliformes from a suction-feeding elopomorph ancestor. As behavioural data on feeding in eels are rare, we used the length of teeth and shape of the mouth opening as morphological proxies to infer that within our sample, 32 eel species bite and 27 use suction to capture prey (see Methods and Supplementary Table 1 ). We note that divergent states in these traits are considered adaptive for biting (long teeth and notched mouth openings) and suction (short teeth and rounded mouths), and morphologically inferred feeding modes for 13 species are corroborated by observations of feeding in the lab ( Supplementary Table 1 ) or by video analysis of prey capture in live animals [34] . Stochastic character mapping of feeding mode on a sample of phylogenetic reconstructions for Elopomorpha revealed that the most recent common ancestor of Anguilliformes was more likely to be a biter (Bayesian posterior probability=0.69) than a suction feeder. Multiple reversions to suction feeding occurred subsequently (mean=14 transitions, 95% credible interval=(3, 33)) and many secondary transitions occurred back to biting (mean=16 transitions, 95% credible interval=(8, 29); see Supplementary Fig. 1 ). Under the alternative scenario—the ancestral eel was a suction feeder (Bayesian posterior probability=0.31)—many transitions between biting and suction feeding were also inferred within Anguilliformes (number of transitions from suction feeding to biting: mean=16, 95% credible interval=(7, 27); number of transitions from biting to suction feeding: mean=18, 95% credible interval=(7, 32)). This complex evolutionary history of feeding mode within eels provides a robust framework for evaluating the differential effects of suction feeding and biting on skull evolution, because distantly related lineages that share the same feeding mode likely vary in background biological traits that can confound comparisons of skull diversification. Morphospace occupation in suction feeders and biters We focused on skeletal elements comprising anterior, ventral and lateral aspects of the oral cavity—the jaws, hyoid apparatus and opercular series—that have been shown to act as ‘mechanical units’ (that is, suites of structurally and mechanically connected bones that move together [37] ) during feeding [24] , [25] , [26] . To quantitatively compare cranial morphological diversity (that is, disparity) between suction feeders and biters, we constructed a morphospace whose axes are the first principal component (PC) of size-corrected trait values for structures comprising each of the three mechanical units ( Fig. 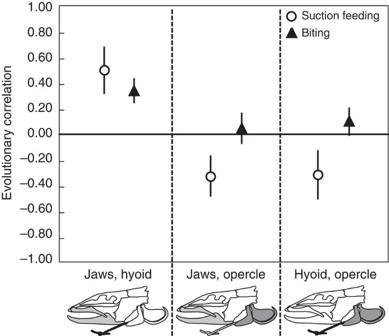Figure 2: Estimates of evolutionary correlations between mechanical units in suction feeders and biters. Error bars are 95% confidence intervals, representing uncertainty in parameter estimation and phylogenetic and ancestral state reconstruction. 1 and Supplementary Table 2 ). We refer to this morphospace as a ‘cranial morphospace’; however, note that unmeasured aspects of the cranial skeleton may show different patterns of disparity in suction feeding and biting eels. Figure 1: Mechanical unit morphological space for 59 anguilliform and 3 other elopomorph species. Axes are the first PCs of phylogenetically controlled interspecific correlation matrices within mechanical units. Axis labels describe the direction of loadings for the morphological variables. Biting species are black triangles and suction feeders are circles; white circles are eels and grey circles are non-anguilliform elopomorphs. Skull images, which have been scaled to the same geometric mean skull size, display a sample of diversity of suction feeding ( a–d ) and biting species ( w–z ) across this morphospace. Skulls have been cleared and stained for bone (red) and cartilage (blue). Species identities are as follows : (a) Heteroconger hassi , (b) Conger myriaster , (c) Anguilla japonica , (d) Ophichthus zophochir , (w) Bathyuroconger vicinus , (x) Morigua javanica , (y) Gymnothorax kidako , (z) Oxyconger leptognathus . Inset shows bones of the jaws (light grey shading), hyoid (dark grey) and opercular series (intermediate grey) on a line drawing of an Anguilla rostrata skull. Abbreviations of bone names are as follows: D, dentary; Mx, maxilla; PMx-Et-V ,premaxillo-ethmo-vomer; BBr, basibranchial; Hy, hyoid; Op, opercle; POp, preopercle; SOp, subopercle. Full size image The first PCs for the jaw and hyoid explain 35.5% and 44.3%, respectively, of the total morphological variance among species within these mechanical units. Biters exhibit values on these morphological axes, indicating a tendency to possess long, gracile jaws and hyoids ( Fig. 1 ). Suction feeders, by contrast, possess shorter and deeper jaws and hyoids, only rarely exhibiting large positive values for either oral jaw or hyoid PC 1 ( Fig. 1 ). Opercular series PC 1 explains 51.3% of the total variance among species and represents the size of the operculum relative to the rest of the skull. Biters show wide variation among species on this axis, whereas most suction feeders have intermediate values and the among-species variability is relatively low ( Fig. 1 ). Compared with suction feeders, biters show greater proper variance (PV)—a metric of disparity that accounts for both variance among species and the strength of covariance between morphological axes [38] —by more than a factor of three (PV bite =9.10±1.14, PV suction =2.80±0.34). Although this metric provides a quantitative way to compare the extent of diversity among extant species, it ignores the influence of shared evolutionary history among them, which may confound apparent variance and covariance among species [39] , [40] . To evaluate feeding mode’s effect on morphological evolution, we used reconstructions of phylogenetic and feeding mode history as the basis for estimating different evolutionary rate matrices for mechanical units (that is, the multivariate pattern of evolutionary change based on a Brownian motion model of evolution) in suction feeders and biters [36] . Patterns of diversification of cranial mechanical units Evolutionary correlations between all pairs of skull mechanical units are stronger (that is, their magnitudes are greater) in suction feeders than biters (Welch’s two-sample t -tests with n suction =30 and n bite =32; jaws—hyoid: t =1.82, df =43.4, P =0.038; jaws—opercular series: t =4.40, df =54.9, P <0.001; hyoid—opercular series: t =4.09, df =46.0, P <0.001; see Fig. 2 ). In fact, in biters the correlation between the jaws and opercular series is not different from zero ( t -tests with n =32: r =0.03±0.05, t =0.67, df =30, P =0.51) and the correlation between the hyoid and opercular series is only marginally greater than zero ( r =0.10±0.04, t =2.14, P =0.041). The jaws and hyoid are, however, significantly correlated during evolution in biters ( r =0.34±0.05, t =6.57, df =30, P <0.001), even though the association is weaker than in suction feeders. Figure 2: Estimates of evolutionary correlations between mechanical units in suction feeders and biters. Error bars are 95% confidence intervals, representing uncertainty in parameter estimation and phylogenetic and ancestral state reconstruction. Full size image Despite differences in the strength of evolutionary correlations among mechanical units, we found little evidence that biters and suction feeders experience different rates of evolution within units (Welch’s two-sample t -tests with n suction =30 and n bite =32; jaws: t =0.09, df =39.5, P =0.47; hyoid: t =0.14, df =34.3, P =0.45; opercular series: t =0.01, df =52.3, P =0.50; see Fig. 3 ). 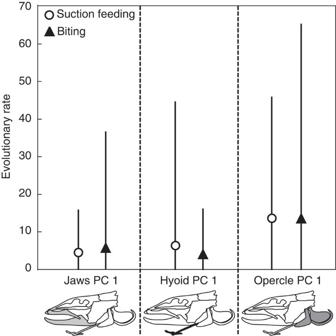Figure 3: Estimates for rates of evolution within mechanical units in suction feeders and biters. Error bars are 95% confidence intervals, representing uncertainty in parameter estimation and phylogenetic and ancestral state reconstruction. Figure 3: Estimates for rates of evolution within mechanical units in suction feeders and biters. Error bars are 95% confidence intervals, representing uncertainty in parameter estimation and phylogenetic and ancestral state reconstruction. Full size image To show that these patterns of diversification are representative of individual skeletal elements, we repeated comparisons of evolutionary correlations and rates using the original morphological traits that make up each mechanical unit (see Methods). Although PC analysis (PCA) allowed us to reduce the dimensionality of our data set, the resulting PCs are linear combinations of covarying traits dependent on the sample of species in the analysis and cannot be interpreted as actual structural features [41] . Nevertheless, results based on each mechanical unit PC 1 reliably summarize differences in evolutionary correlations and rates for individual morphological traits. The magnitudes of correlations between traits from different mechanical units are generally greater in suction feeders than in biters with only two exceptions (the correlations between lower jaw opening in-lever and hyoid and between lower jaw closing in-lever and the operculum), and the differences between feeding modes tend to be largest for correlations involving traits that make up the operculum ( Supplementary Figs 2–4 ). In addition, rates of evolution tend to be similar for most morphological traits, but when rates do differ they are not consistently higher for either feeding mode ( Supplementary Figs 2–4 ). Within- versus between-mechanical unit integration Comparisons of the overall strength of evolutionary integration (that is, the mean magnitude of correlations) between mechanical units relative to evolutionary integration within units revealed different patterns in suction feeders and biters ( Fig. 4 ). In suction feeders, the strength of between-mechanical unit integration does not differ from within-unit integration (Welch’s two-sample t -tests with n within =n between =30; jaws: t =1.37, df =42.1, P =0.18; hyoid: t =0.28, df =50.4, P =0.78; opercular series: t =0.02, df =48.2, P =0.99). In biters, however, between-mechanical unit integration is weaker than the integration within the opercular series (Welch’s two-sample t -tests with n within =n between =32: t =3.44, df =39.7, P =0.001), stronger than within the hyoid ( t =2.66, df =51.0, P =0.011) and no different from integration within the jaws ( t =1.19, df =39.7, P =0.24). Moreover, we found that feeding modes exhibit similar strengths of integration within the jaws (Welch’s two-sample t -tests with n suction =30 and n bite =32; t =0.03, df =43.6, P =0.49) and within the opercular series ( t =0.37, df =40.7, P =0.36) but differ in integration within the hyoid ( t =4.39, df =32.6, P <0.001), with biters showing weaker overall correlation ( r bite =0.16±0.02; r suction =0.37±0.04). We note that similarity between feeding modes in the strength of integration within mechanical units, as we have quantified it here, does not imply similarity in the correlation matrices, only that the overall magnitude of integration is similar. 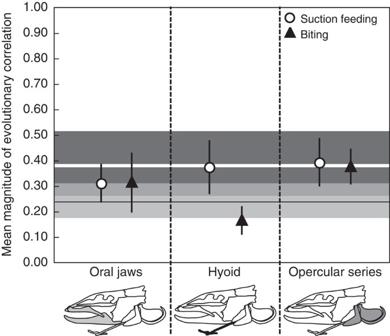Figure 4: Evolutionary correlations within- versus between-mechanical units in suction feeders and biters. Shapes are estimates for the mean magnitudes of evolutionary correlations within mechanical units for suction feeders (circles) and biters (triangles). Error bars are 95% confidence intervals. Thick horizontal lines are the mean magnitudes of evolutionary correlations between-mechanical units (white is suction feeding and black is biting) and shaded regions represent their 95% confidence intervals (dark grey is suction feeding and light grey is biting). Figure 4: Evolutionary correlations within- versus between-mechanical units in suction feeders and biters. Shapes are estimates for the mean magnitudes of evolutionary correlations within mechanical units for suction feeders (circles) and biters (triangles). Error bars are 95% confidence intervals. Thick horizontal lines are the mean magnitudes of evolutionary correlations between-mechanical units (white is suction feeding and black is biting) and shaded regions represent their 95% confidence intervals (dark grey is suction feeding and light grey is biting). Full size image We show that historical transitions between prey-capture behaviours, inferred by changes in the shape of the mouth opening and tooth morphology, correspond to shifts in evolutionary integration of the skull. Prey capture by biting requires less behavioural coordination among the jaws, hyoid and opercular mechanical units compared with suction feeding [34] , and transitions to biting in eels are associated with weakening of evolutionary correlations between mechanical units ( Fig. 1 ). Our results therefore support the hypothesis that relaxed functional integration has allowed biters to evolve a greater diversity of mechanical unit combinations compared with suction feeders and to ultimately occupy a wider expanse of cranial morphospace ( Fig. 1 ). Conversely, greater evolutionary integration in suction feeders suggests that their cranial diversification has been constrained by the between-mechanical unit coordination that is required to maintain an anterior-to-posterior wave of oral cavity expansion [24] , [27] , [29] . Although our results support the hypothesis that the strength functional integration shapes evolutionary integration, we note several caveats. First, our phylogenetic comparative approach is by nature correlative and precludes testing whether shifts in functional integration cause shifts in evolutionary integration. Instead, we document an association between reconstructed feeding behaviour and evolutionary integration that is consistent with a causal hypothesis. Second, for the majority of eel species in our data set, we lack feeding behavioural data and instead use morphology to infer modes of prey capture. We assume that divergent morphological states reflect suction feeding and biting prey capture, and note that empirical data for a subset of eels support this assumption. Third, we are unable to determine the exact sequence of anatomical and functional changes that occur during transitions between feeding modes. Instead of attempting such detailed reconstructions, we assume that transitions in feeding behaviour and functional integration are tightly linked. We note that this assumption is firmly grounded in the results of prior functional studies [34] (also see Methods). Our results suggest that functional integration can play an important role in driving one of the most intriguing patterns in macroevolution: some combinations of morphological traits are very common, resulting in regions of morphospace that are populated with many species, but other combinations are rare, leading to large areas of sparsely occupied morphospace [42] , [43] . We propose that strong functional integration, such as that imposed by suction feeding, can limit the combinations of trait values that are permitted to evolve, resulting in densely packed regions of morphospace. However, the weakening of functional integration following the origin of a novel behaviour, such as biting, releases constraints and allows new combinations of traits to evolve, leading some species to reach previously unoccupied areas of morphospace. In the case of eels, biters have diversified to take on skull morphologies that are not seen in suction feeders. In particular, most biters possess elongated jaws with sharp, recurved teeth and slender hyoids, and vary extensively in opercular series morphology. However, suction feeders share similar robust jaws and hyoids, and are limited to relatively large opercula ( Fig. 1 ). The functional and evolutionary linkages between the jaws, hyoid and opercular series in suction feeders indicate that together these mechanical units can be considered an evolutionarily stable configuration, a suite of structures bound by internal selection on functional output [3] , [4] . Suction-feeding eels and other elopomorph fishes provide an empirical example of the evolutionarily stable configuration model prediction that functional relationships between structures limit the possibilities of morphological diversification. However, despite the strong effect of feeding mode on evolutionary integration, our results do not support the prediction that integration limits the rate at which morphological differences accumulate among species [1] , [3] , [4] , [17] . We find no evidence that suction feeders and biters experienced different rates of mechanical unit diversification ( Fig. 3 ). Our results, therefore, suggest the possibility that shifts in the strength of evolutionary integration can occur independently of changes in evolutionary rates. However, we also note that the absence of a statistical difference in rate between feeding modes may be partly a consequence of high variance in our estimates of evolutionary rates, which results from a combination of phylogenetic uncertainty, uncertainty in the reconstruction of feeding mode on the tree and variance in the estimated parameters conditioned on any particular phylogeny and feeding mode reconstruction. Increased power to identify a rate difference, if one exists, could result from the addition of new phylogenetic data or species, or by using a more complex model for feeding mode evolution that permitted feeding-mode state-dependent diversification on the tree [44] . With that in mind, however, our current results suggest that if rate differences exist between feeding modes for the characters in our study, they are probably relatively small. Similarity in rates of mechanical unit evolution may still be consistent with the hypothesized constraining effects of tight functional integration in suction feeders. If some suction-feeding eel species re-acquired this feeding mode from biting ancestors, which had diversified into disparate regions of morphospace ( Fig. 1 and Supplementary Fig. 5 ), secondary transitions to suction feeding would have involved strong selection and rapid evolution towards suction-adapted skulls from widely dispersed biting morphologies. This scenario is supported by the relatively restricted region of morphospace occupied by both non-anguilliform elopomorphs and suction-feeding eels ( Fig. 1 ). Alternatively, rate similarity across behavioural transitions could be a consequence of parallel extrinsic selection associated with diet diversification. Suction feeding and biting eels are thought to feed on similar functional prey categories, including evasive prey (for example, fish and squid) and substrate-associated prey (for example, crabs) [35] , [45] , [46] . Suction-feeding and biting eels may have diversified between long, gracile jaws and skulls to enhance feeding on evasive prey and short, robust forms to capture and process attached prey, as suggested by the spread of both suction-feeding and biting species on jaws PC 1 and hyoid PC 1 ( Fig. 1 ). Our results further suggest that functional integration can cause evolutionary correlations between separate mechanical units that are as strong as that within units ( Fig. 4 ). Strong between-unit correlations may arise, because the jaws, hyoid and opercular series make up the oral cavity, which acts as a single functional unit (that is, a suite of structures or mechanical units united by shared function [3] , [37] , [47] ) whose expansion is critical to generating the water flow that entrains suction feeders’ prey [29] . Even though the jaws, hyoid and operculum are mechanically capable of independent movements relative to one another, the functional demands of suction feeding limit their actual kinematics to a set of tightly coordinated stereotypical movements [25] , [28] , [29] . Relaxed functional integration among skeletal elements is thought to allow novel and extreme morphologies to arise [1] , [3] , [16] , [18] , [19] , [20] , and indeed this is the case following the evolution of biting in eels. In general, the hyoids of biting species are more slender than those of suction feeders, but some biting species have evolved highly reduced, non-functional hyoids ( Fig. 1 ), in which within-unit evolutionary integration has degraded ( Fig. 4 ). This extreme morphology is also associated with a more specialized biting behaviour. Whereas many biters retain the ability to generate suction for transporting prey from the jaws to the oesophagus [48] , biters that exhibit severe hyoid reduction, such as moray eels, possess little or no capacity to generate suction [34] . Morays show no detectable hyoid depression during feeding strikes, the hyoid is not involved in mouth opening and the pectoral girdle, an attachment site for the main hyoid retractor muscle (the sternohyoideus) [25] , is also reduced [34] . This specialized mode of biting expands the variety of skull morphologies biting eels exhibit, as species with uniformly reduced hyoids, such as the morays, experience adaptation of the jaws to divergent diets and prey-capture strategies—such as crushing hard prey, snatching elusive prey or biting off pieces of large prey [35] , [49] . These patterns suggest that by allowing extreme forms to evolve, weakened functional integration can further enhance the variety of morphological combinations found among species. Disruption of integration can also facilitate functional innovation, as structures are able to respond in new ways to selection for other functions. For example, the weakened cranial integration we found in biters may have allowed a novel gill-ventilation mechanism to evolve. Most teleosts, including non-anguilliform elopomorphs and many eels, ventilate their gills using a coupled buccal-opercular pump that requires coordinated hyoid and opercular movements to transport water through the buccal and opercular cavities [50] , [51] . In moray eels, however, the buccal pump is dominant and the opercular series is highly reduced. Water moves from the buccal cavity to a parabranchial chamber that houses the gills and exits through reduced circular openings formed by flaps of skin, rather than through a large opercular bone that abducts. Unlike the buccal-opercular pump, the buccal-parabranchial pump requires little coordination between the hyoid and opercular series, and this derived gill ventilation mechanism in morays may reinforce the weak evolutionary correlation we observe within biting eels. Altogether, our results show that behavioural transitions can spur morphological diversification by altering the strength of functional integration among structures. Although relaxed functional integration is necessary to allow for greater evolutionary independence among structures, it alone is insufficient to drive diversification. The underlying genetic architecture and developmental connections must also allow for novel morphological combinations. In addition, extrinsic natural selection is necessary to push species to disparate regions of morphospace. Selection for diverse morphologies may follow directly from behavioral transition if the new behaviour allows access to new resources [52] . However, as they can change the strength of functional integration among structures, we speculate that behavioural transitions can fundamentally alter the adaptive landscape even in the absence of concomitant shifts in resource use (also see Walker [14] ). We therefore propose that behavioural transitions, through their effects on functional integration, play an important role in explaining shifts in the pattern and process of morphological diversification across the tree of life and urge further investigation into the connection between functional relationships and phenotypic evolution. Details on the functional integration of suction feeding and biting Successful suction feeding requires rapid and highly coordinated movements of cranial skeletal elements to increase oral cavity volume and generate water flow strong enough to carry prey into the mouth [24] , [25] , [26] . We focused on three mechanical units comprising anterior, ventral and lateral aspects of the oral cavity—the jaws, hyoid and opercular series. Although other mechanical units and structures are involved in prey capture, we examined these three mechanical units because their movements are well characterized and known to be important to suction generation [24] , [25] , [26] , [27] , [28] , [29] . A stereotypical temporal progression of jaw opening, hyoid depression and opercular flaring creates an anterior-to-posterior wave of oral cavity expansion (see Supplementary Fig. 5 ), which is mechanically essential for maintaining a unidirectional flow of water into the mouth and through the buccal cavity [27] , [29] . In fact, the pattern of movements of mechanical units involved in oral expansion is strongly conserved among a phylogenetically diverse array of teleost fish species [25] , [28] . Rather than rapid oral cavity expansion, the prevailing functional demand of biting is forceful contact between the jaws and prey [30] , [31] , [32] . Feeding kinematics reflect this functional demand. Unlike the rapid, stereotypical strike of suction feeders, skull movements are slower [33] , [34] and more variable from strike to strike in individual biters than they are in suction feeders, as biters modulate jaw position to close firmly onto their prey [34] (see Supplementary Fig. 5 ). The demonstrated difference between suction feeding and biting in the strength of functional integration among mechanical units provides a firm empirical foundation for using reconstructions of feeding behaviour to infer historical changes in the strength of functional integration. Quantifying mechanical unit morphology For each of 59 anguilliform and three other elopomorph species, we measured skeletal elements comprising the jaws, hyoid and opercular series. Specimens were obtained from personal or museum collections, including the Museum of Comparative Zoology and the California Academy of Sciences, and were cleared and double stained for bone and cartilage to reveal internal skeletal anatomy [53] . We measured seven traits of the jaws (dentary length and depth, lower jaw closing in-lever, lower jaw opening in-lever, maxilla length, premaxillo-ethmo-vomerine (PMx-Et-V) length and width), three hyoid traits (basibranchial length, hyoid length and hyoid depth) and four aspects of the opercular series (opercle length, opercle depth, subopercle length and preopercle length). In addition, we measured skull length, width and depth, and took the geometric mean of these dimensions as a measure of skull size, which we used to size-correct morphological trait values (see below). We obtained all measurements in mm using analog calipers or a Leica M60 fitted with an ocular micrometer. We sampled multiple individuals per species for all but eight species (median=2 individuals; range=1–4), and evaluated species mean values of morphological measurements from individuals (morphological data for individual specimens are available in the Dryad Digital Repository: http://dx.doi.org/10.5061/dryad.32r3q ). To account for morphological variation among species that results from differences in size, we regressed log-transformed species means for morphological variables against the log-transformed geometric mean of skull dimensions and took residuals as size-corrected species values. We used the geometric mean of skull dimensions for size correction rather than overall body size (for example, standard length), because the former exhibits a much stronger relationship with cranial skeletal elements. We used generalized least squares regression implemented in phyl.resid of the phytools package [54] , [55] for R [56] , to account for non-independence among species resulting from phylogenetic relatedness. We reduced the dimensionality of morphological variation in each mechanical unit using PCA. Comparisons of evolutionary correlations and rates between suction feeders and biters for all individual traits would be computationally prohibitive; a model including separate rates and covariances in suction feeders and biters would involve 210 parameters based on data for 13 traits in 62 species (see ‘Comparing evolutionary correlations and rates’ below). Instead, we reduced the dimensionality of each mechanical unit from a suite of traits to its first PC, which is the linear combination of morphological variables corresponding to the primary axis of variation and covariation among species. We used the function phyl.pca in the phytools package [54] , [55] for R [56] , to perform PCA on the correlation matrix of species values in a manner that accounts for similarity resulting from phylogeny. We performed phylogenetic PCA analysis separately for each mechanical unit and used species scores for each PC 1 as species values for mechanical unit morphology (see Supplementary Table 2 ). Reconstructing phylogenetic and feeding-mode history We estimated phylogenetic relationships among 119 anguilliform species and 5 other elopomorph species based on sequences for three mitochondrial genes ( 12S , 16S and Co1 ) comprising 2945 base pairs. We downloaded published sequences [57] , [58] , [59] from GenBank with the following accession numbers: 12S: DQ645647-DQ645685 and AF454707-AF455759 ; 16S: DQ645686-DQ645727 and AF455760-AF455783 ; CO1: AP010840-AP010870 , NC_013601 and NC_013602 . We assembled alignments for each gene region by observing with the naked eye and manually removed ambiguously alignable regions from 12S and 16S matrices. We used Bayesian methods and a relaxed molecular clock [60] implemented in the computer programme BEAST [61] to infer phylogenetic relationships and branch lengths in relative time. We used the General Time Reversible model of sequence evolution with gamma distributed among-site rate variation and invariant sites. Rate variation among phylogenetic branches was approximated by an uncorrelated lognormal distribution with mean rate specified as 1.0 (that is, no absolute time calibration). To estimate the posterior probability distribution of trees and model parameters, we ran BEAST’s Markov Chain Monte Carlo algorithm [61] 5 times for 50 million generations each. For each run, the starting tree was randomly generated according to a Yule (pure-birth) process, the first five million generations were discarded as burn-in and chain states were sampled every 5,000 generations. We used the computer programme TRACER [61] to confirm adequacy of effective sample sizes for the combined posterior sample of trees and model parameters [60] . To incorporate uncertainty in phylogeny reconstruction into estimation of evolutionary rates and correlations, we retained a subsample of 1,000 trees for use in subsequent analyses (sequence alignments and maximum clade credibility tree available in TreeBase: study accession number S16413). Each of these trees was pruned to include only the 62 species in our morphology data set. We assigned feeding-mode states (biting or suction) to all species in our morphological data set. As information on prey capture behaviour in eels is limited, feeding mode was determined by examining a suite of morphological traits that are well known to differentiate biters from suction feeders [26] , [62] , [63] . To avoid circularity in our analysis, we scored four discrete cranial traits that do not overlap with the skeletal elements measured as part of our main analysis: oral teeth, PMx-Et-V teeth, hyomandibular orientation and mouth shape. Oral teeth are either short (scored as 0) or long (scored as 1). Oral teeth of suction feeders are generally short, because prey are ingested without contacting the jaws and long teeth can interfere with prey capture by suction, whereas possession of long, pointed teeth indicates prey are ensnared by biting. Teeth on the PMx-Et-V are absent (=0), short (=1) or long (=2). Similar to oral teeth, long PMx-Et-V teeth indicate use in biting prey. In both cases, teeth were considered long when they were >1 mm. The hyomandibula articulates with the lower jaw and is oriented anteriorly (0), vertically (1) or posteriorly (2). Posteriorly oriented hyomandibulae accommodate longer lower jaws, typically present in biters, and often result in lateral notches in the mouth opening. The mouth opening is rounded (0), semi-rounded (1), notched (2) or deeply notched (3). A rounded opening is critical to directing water flow in front of the mouth, while lateral notches make suction production much less efficient [26] , [62] , [63] . The degree of roundedness or notching is obvious in lateral view when the mouth is fully opened. The mouth is made round and flat (perpendicular to the direction of water flow) by lateral abduction of the lower jaw, downward rotation of the maxilla, and stretching of membranous connective tissue that runs between the lower jaw and maxilla. The opening is considered only semi-rounded when slight notches are present but lateral abduction of the lower jaw and rotation of the maxilla still occur. Notched mouths exhibit reduced connective tissue layers, little lateral rotation of the lower jaw and negligible maxilla movement, which expose gaps in the sides of the mouth opening. Deeply notched mouths exhibit the most extreme lateral gaps. For all four characters, the numerical scores for trait states are ordered such that higher values indicate adaptation for biting. By adding the scores for all characters, we obtained a bite score for each species. In general, species with bite scores of three or below had short oral teeth, no or short vomerine teeth, anteriorly oriented or vertical hyomandibulae and rounded or semi-rounded mouths. We classified these species as suction feeders. Biters on the other hand, had bite scores >3 and exhibited variable teeth, posteriorly oriented or vertical hyomandibulae, and notched or highly notched mouths. Feeding-mode assignments based on this scoring scheme are consistent with personal observations of feeding behaviour for 13 species, including species with intermediate bite scores of three and four (see Supplementary Table 1 ). Given assigned states in elopomorph species, we used stochastic character mapping [64] to reconstruct ancestral feeding mode on each of the 1,000 pruned trees sampled from our phylogenetic analysis (see Supplementary Fig. 1 ). We implemented this method in the phytools [55] function make.simmap using a transition rate matrix sampled from the posterior probability distribution using Bayesian Markov Chain Monte Carlo. We used a gamma prior probability distribution on the rate with β set to 2.0 and empirically determined α (that is, we set α to the product of β and the empirical mean for the transition rate). We sampled one stochastic map per phylogenetic tree, resulting in 1,000 reconstructions of feeding mode. Iterating analyses across this sample allowed us to integrate over uncertainty in both phylogeny and ancestral state estimation. Comparing evolutionary rates and correlations To evaluate whether transitions in feeding mode lead to shifts in patterns of morphological diversification, we fit separate evolutionary correlations and rates to species values for mechanical unit morphology (that is, species scores for mechanical unit PC 1) given reconstructions of feeding mode and phylogeny. We used the method of Revell and Collar [36] , which allowed us to estimate the evolutionary rate matrix or matrices for mechanical unit PC 1 assuming a Brownian motion model of evolution. The evolutionary rate matrix contains the evolutionary rates (instantaneous variances of the Brownian process) for each character on the diagonal and evolutionary covariances between characters elsewhere. Evolutionary correlations are derived from these estimated rates and covariances. We fit a two-matrix model, which allows separate evolutionary rate matrices for lineages inferred to be suction feeding and biting according to feeding-mode reconstructions. We also fit a single-matrix model in which only one evolutionary rate matrix is estimated for all elopomorph lineages regardless of feeding mode. We performed model fitting using maximum likelihood implemented in the function evol.vcv of phytools [36] , [54] and iterated over the sample of 1,000 feeding-mode reconstructions. This procedure resulted in a distribution of likelihood scores and parameter estimates for each model. We compared fit of the two models for each reconstruction using the small sample size corrected Akaike Information Criterion (AIC) and assessed model preference based on corrected AIC and Akaike weight (AICw) [65] . Comparisons of fit revealed support for both the one- and two-matrix models based on mean weight (AICw(one-matrix)=0.56±0.44; AICw(two-matrix)=0.44±0.44) and we found model preference varied across trees (the two-matrix model was preferred in 44.6% of reconstructions; see Supplementary Fig. 6 ). To estimate model parameters given the uncertainty in model preference, we evaluated the mean of parameters estimated for the one- and two-matrix models weighted by their Akaike weights [65] . For each feeding-mode reconstruction, we estimated model averaged evolutionary rates and covariances in suction feeders and biters, and evaluated Pearson correlation coefficients from these values. We then computed the mean model averaged rates and correlations across reconstructions for suction feeders and biters. We used Welch’s t -test [66] to assess the statistical significance of differences between suction feeders and biters in evolutionary rates and correlations. The variances of parameter estimates—calculated separately for suction feeders and biters—were the sums of two independent sources: variance in parameter estimation and variance resulting from variable phylogeny and feeding-mode reconstructions. Computing the total variance in parameter estimation this way assumes only that variation from the two sources is uncorrelated and will be conservative if they are correlated. For each reconstruction, we obtained variance in estimation for all parameters of the one- and two-matrix models using the evol.vcv function of phytools [54] and calculated the model-averaged estimation variance for all parameters. We then evaluated the overall estimation variance as the mean variance across reconstructions. Variance in parameter estimates resulting from phylogenetic and ancestral state uncertainty was calculated from the distribution of model-averaged rates and correlations across reconstructions. Degrees of freedom were calculated based on Welch–Satterthwaite equation [66] , [67] , with sample sizes equal to the number of species in each feeding-mode category. The method we used to fit one and two rate matrix models did not account for trait variation within species, which could bias estimates of evolutionary rates and correlations [68] , [69] , [70] . To investigate the effects of within-species variation on our results, we compared pooled within-species s.d. and correlations in suction feeders and biters (see Supplementary Methods ). Overall, we found that within-species variation was small relative to between-species differences. In suction feeders, the ratio of between-species to within-species variance is 6.5 for jaws PC 1, 7.2 for hyoid PC 1 and 8.1 for opercular series PC 1, and in biters these ratios are equal to 12.6 (jaws), 10.4 (hyoid) and 11.4 (opercular series, also see Supplementary Table 3 ). In addition, we found that within-species correlations between mechanical units were negligible, except for the correlation between the hyoid and opercular series in suction feeders ( Supplementary Table 3 ). Numerical simulations using a Brownian motion model of evolution show that the observed level of within-species variation and correlation generates minimal bias in evolutionary rate and correlation estimation ( Supplementary Methods and Supplementary Figs 7 and 8 ). To evaluate whether comparisons of evolutionary rates and correlations for mechanical unit PC 1s are representative of those for individual morphological traits, we conducted a modified version of the analysis described above using the original morphological variables. As noted above (see Methods, ‘Quantifying mechanical unit morphology’), we were unable to simultaneously estimate separate rates and covariances in suction feeders and biters for all morphological variables. Instead, to reduce the dimensionality of the data set, we randomly selected one trait from each mechanical unit and estimated model-averaged evolutionary rate matrices for suction feeders and biters. We carried out this procedure over all 1,000 trees, sampling new traits within mechanical units for each tree, and obtained distributions of rates and magnitudes (that is, absolute values) of between-mechanical unit correlations for all morphological traits. Note that between-unit correlations for each individual trait include estimates between the focal trait and all traits comprising the other mechanical units (for example, the correlation between dentary length and the hyoid includes estimates between dentary length and each of the three hyoid characters—basibranchial length, hyoid length and hyoid depth). As the directions of correlations involving different traits can differ (for example, dentary length by hyoid length versus dentary length by hyoid depth), it was necessary to average over correlation magnitudes rather than magnitudes and directions. Moreover, the spread of between-unit correlations is a function of both variation in estimates involving different traits and variation in estimates across trees. In addition, we note that estimates of rates and correlations for each morphological trait are based on a fraction of trees (approximately equal to 1/the total number of traits within the mechanical unit). Between- versus within-mechanical unit integration Within both suction feeders and biters, we compared the overall magnitude of evolutionary integration between mechanical units to the level of evolutionary integration within them. We evaluated integration between mechanical units as the mean of the absolute values of their three evolutionary correlations, following Young and Hallgrimsson [11] . Integration within a mechanical unit was determined as the mean magnitude of evolutionary correlation between morphological traits within that unit, where the pairwise evolutionary correlations between traits were estimated using a model-fitting and model-averaging approach similar to the method described above. We reduced the number of morphological variables within a mechanical unit by randomly sampling three traits from within it (except the hyoid, which contained only three morphological traits). Sampling a new set of traits for each of 1,000 trees resulted in correlation estimates for all combinations of traits. We used Welch’s t -test [66] (as described in the previous section) to compare mean correlations at two levels: (1) within-mechanical unit versus between-mechanical unit and (2) within-mechanical unit in suction feeders versus biters. How to cite this article: Collar, D. C. et al . Biting disrupts integration to spur skull evolution in eels. Nat. Commun. 5:5505 doi: 10.1038/ncomms6505 (2014).